Revealing the ultrafast process behind the photoreduction of graphene oxide Effective techniques to reduce graphene oxide are in demand owing to the multitude of potential applications of this two-dimensional material. A very promising green method to do so is by exposure to ultraviolet irradiation. Unfortunately, the dynamics behind this reduction remain unclear. Here we perform a series of transient absorption experiments in an effort to develop and understand this process on a fundamental level. An ultrafast photoinduced chain reaction is observed to be responsible for the graphene oxide reduction. The reaction is initiated using a femtosecond ultraviolet pulse that photoionizes the solvent, liberating solvated electrons, which trigger the reduction. The present study reaches the fundamental time scale of the ultraviolet photoreduction in solution, which is revealed to be in the picosecond regime. Graphene was discovered less than a decade ago [1] and has attracted an enormous amount of attention owing to its peculiar properties (electrical [1] , [2] , [3] , optical [4] , structural [5] and so on). The study of graphene and its use for practical applications has given birth to a parallel research field concerning the chemistry of graphene and its derivatives [6] , [7] , [8] , [9] . However, large-scale single layers of pristine graphene are challenging to obtain using conventional methods (mechanical exfoliation, epitaxial growth, CVD and so on), and so material scientists are exploring solution chemistry as an alternative path. In particular, much effort is currently focused on the fabrication [10] and reduction of graphene oxide (GO) in an attempt to produce high-quality graphene in solution or in solid state. This method is extremely attractive because GO is soluble in water and can easily be produced in large quantities (for example, by the Hummers and Offeman [11] and Staudenmaier [12] methods). Understanding the reduction process is not only of importance from a fundamental point of view but is also key to the improvement and exploitation of reduced GO (rGO) on industrial scales. Over the years, various procedures have been reported; the reactions range from the widely used sodium borohydride [13] and hydrazine [14] , [15] methods to catalytic [16] , plasma-induced [17] , thermally induced [18] , [19] , [20] and photoinduced reduction [21] , [22] , [23] . Although each of these methods has its own merits, light-induced reduction of GO promises to be a rapid and facile way of producing rGO while avoiding the use of harsh chemicals. Pioneering work [21] , [24] , [25] , [26] , [27] on the photoreduction deduced a reaction time scale that ranged from 600 μs [23] up to hours [26] . This literature provides a variety of recipes with a broad range of wavelengths, exposure times, light intensities and environments (solids and liquids). Such exposure to light can induce thermal or direct reduction, but can also affect the environment leading to indirect reduction. Distinguishing between the possible reduction mechanisms and understanding their dynamics is challenging but is important from both a fundamental and applied point of view. Herein we investigate the nature of the ultraviolet photoreduction of GO in solution by using femtosecond laser pulses in a pump–probe fashion. A flowing water dispersion of GO is irradiated by an ultraviolet femtosecond pulse (the pump), followed by a second femtosecond visible pulse (the probe). Varying the delay between the arrival of the pump and the probe enables the observation of the evolution of the reaction in real time. Our results corroborate a recently proposed model [28] for GO photoreduction in water: the ultraviolet light (4.6 eV) is absorbed by the solvent through a nonlinear process, namely two-photon absorption. This process excites the water above its photoionization threshold (6.5 eV) leading to the generation of solvated electrons [29] , which are then responsible for the production of rGO. The entire reduction dynamics are unveiled by transient absorption measurements and are found to occur on a picosecond time scale. These observations demonstrate that the ultraviolet reduction is ultrafast and involves the intermediacy of solvated electrons to drive the reduction step. In the following discussion, we will explain why this seemingly unlikely process needs to be invoked and we will confront this model with other potential photoreduction pathways like heating or direct photoionization. Production and characterization of rGO A proof-of-principle demonstration of the reduction was made by placing a cell containing a GO dispersion in the path of a femtosecond pulsed ultraviolet laser. Depicted in the inset of Fig. 1a , a 1-mm thick vial of 0.5 mg ml −1 of GO in water is shown before and after 30,000 ultraviolet pulses over a 2 cm line (see Supplementary Movie 1 ). At first, the GO dispersion is featureless; after irradiation, a darker line is visible, which suggests that rGO formed owing to the exposure to ultraviolet light. Several methods were used to confirm the identity of the photoproduct. Conventional ultraviolet–visible spectroscopy was performed on the sample before (red) and after (black) photoreduction ( Fig. 1a ). The rGO photoproduct can be distinguished from the GO spectrum by an increase of absorption in the 280–800 nm range that corresponds to the restoration of the π network of the carbon structure [25] . 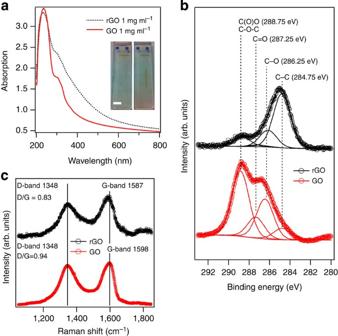Figure 1: Characterization of the reduced graphene oxide. ultraviolet–visible absorption spectra (a) of aqueous dispersions of graphene oxide (GO) (red solid line) and photoreduced GO (black dashed line). Inset (a): photographs of a 0.5 mg ml−1dispersion of GO in water before (left) and after (right) pulsed ultraviolet laser irradiation (scale bar, 5 mm). X-ray photoemission spectra (b) of GO (red, bottom) before and (black, top) after ultraviolet laser irradiation. Raman spectra (c) of GO (red, bottom) before and (black, top) after ultraviolet laser irradiation. Figure 1c displays the Raman spectra from before (red) and after (black) ultraviolet irradiation. One can see for the starting material ( Fig. 1c (red)) the characteristic D- and G-bands at 1,348 and 1,598 cm −1 , respectively, and a D/G intensity ratio of 0.94. The rGO spectrum ( Fig. 1c (black)) shows a slightly shifted G-band peak towards lower values and a reduced D/G intensity ratio of 0.83. This observation, explained by a graphitization of the sample as described by Yang et al . [30] , is in good agreement with the extended literature [17] , [18] , [31] , [32] . However, the D/G intensity depends largely on the quality of the starting GO and the reduction method employed [18] ; therefore, X-ray photoemission spectroscopy (XPS) was used to quantify the degree of reduction. The photoemission spectra of the carbon 1 s line before (red) and after (black) ultraviolet irradiation is given in Fig. 1b . Figure 1: Characterization of the reduced graphene oxide. ultraviolet–visible absorption spectra ( a ) of aqueous dispersions of graphene oxide (GO) (red solid line) and photoreduced GO (black dashed line). Inset ( a ): photographs of a 0.5 mg ml −1 dispersion of GO in water before (left) and after (right) pulsed ultraviolet laser irradiation (scale bar, 5 mm). X-ray photoemission spectra ( b ) of GO (red, bottom) before and (black, top) after ultraviolet laser irradiation. Raman spectra ( c ) of GO (red, bottom) before and (black, top) after ultraviolet laser irradiation. Full size image The removal of the oxygen content after the photoreduction is obvious and observable as a dramatic decrease of the C–O (286.25 eV), C=O (287.25 eV), C–O–C and C(O)O (288.75 eV) peaks, meaning a restoration of the pure C–C bond from 8–66%. One can conclude that the sample produced after ultraviolet irradiation is rGO. Observation of the ultrafast reduction of graphene oxide The core of this work is displayed in Fig. 2 , showing the concentration-dependent transient absorption measurements of GO in water. The reduction was initiated using a 266 nm pump and the differential absorption of a 400 nm probe was monitored at various delay times. As the reduction is irreversible, all of the following experiments were performed with the sample flowing through an optical cell to ensure a continuously refreshed sample. For all concentrations, a steep rising peak followed by a rapid decay (<2 ps, Fig. 2a ) and a slower decay (<250 ps, Fig. 2b ) can be observed. This behaviour is due to multiple contributions from the water and GO. The initial rise corresponds to the excitation of water via two photon absorption and the photo-excitation and ionization of GO. The water-excited state leads [33] to the generation of OH aq , H 3 O + aq and solvated electrons (e − aq ) within 1 ps. Any ionization of GO will likewise generate solvated electrons but this electron source term represents an oxidation step. Only the solvated electrons generated in the water region lead to a net surplus of electrons with respect to the GO valence occupancy that in turn can drive the overall reduction process. The slow decay (for t <250 ps) of the absorption transient results from a decrease in the population of the mobile solvated electrons due to either interaction with GO or recombination with parent ions. 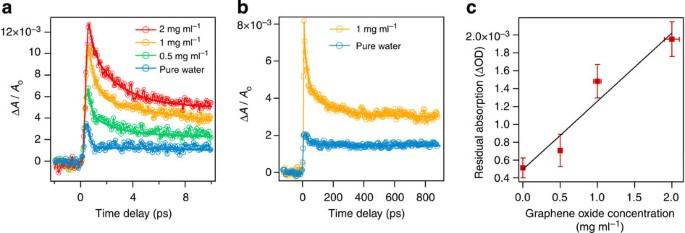Figure 2: Evidence for an ultrafast time scale. Transient differential absorption of ultraviolet-irradiated aqueous graphene oxide (GO) dispersions at 400 nm. (a) Titration of the GO concentration dependence of the dynamics, in water, ranging from 0 mg ml−1to 2 mg ml−1on a 10 ps time scale. (b) Long time scale dynamics of a 1 mg ml−1GO dispersion versus pure water. (c) Plot of the residual absorption value in ΔOD versus graphene oxide concentration. The vertical error bars are the standard deviation of the calculated values displayed. Each point represents the average intensity of the last 2 ps (from 8–10 ps), thus the error bars represent the noise level. The horizontal error bars represent an estimated 5% experimental error on the measure of the absolute GO concentration. The overall reaction is Figure 2: Evidence for an ultrafast time scale. Transient differential absorption of ultraviolet-irradiated aqueous graphene oxide (GO) dispersions at 400 nm. ( a ) Titration of the GO concentration dependence of the dynamics, in water, ranging from 0 mg ml −1 to 2 mg ml −1 on a 10 ps time scale. ( b ) Long time scale dynamics of a 1 mg ml −1 GO dispersion versus pure water. ( c ) Plot of the residual absorption value in ΔOD versus graphene oxide concentration. The vertical error bars are the standard deviation of the calculated values displayed. Each point represents the average intensity of the last 2 ps (from 8–10 ps), thus the error bars represent the noise level. The horizontal error bars represent an estimated 5% experimental error on the measure of the absolute GO concentration. Full size image The data contained in Fig. 2a,b are consistent with this model. The long-lived component of pure water corresponds to a residual Δ A / A 0 of ~1.5 × 10 −3 after 1 ns and is assigned to a fully thermalized species of solvated electrons [34] , [35] , [36] . The increased residual Δ A / A 0 of GO-containing samples, when compared with pure water, results from the additional absorption of newly formed rGO. A quantification of these results was obtained by comparing the residual of the transient absorption with fully rGO absorption extracted from Fig. 1 . This analysis shows a reduction of ~2% after 250 ps. Multiple shots will therefore be necessary to fully reduce the sample. From Fig. 2c , one sees that the final absorption (proportional to the quantity of rGO produced) increases linearly with the GO concentration indicating that the reduction efficiency is concentration independent. Although from the previously discussed results it is already clear that a photo-activated process is present in aqueous GO dispersions, additional time-resolved visible spectroscopy measurements were performed to further confirm the product of the observed photochemical reaction. This technique enables the observation of the variation of the differential absorption Δ A / A 0 over a wide spectrum (590–760 nm) unlike the single wavelength (400 nm) as in Fig. 2a,b . The results of these experiments are displayed in Fig. 3a,b with time ranges of 10 ps and 1 ns, respectively. The GO concentration was 2 mg ml −1 . After time zero, one can observe a strong but spectrally non-uniform change in absorption. Two regions of more intense Δ A / A 0 can be seen, one at low wavelengths (<660 nm) and one at high wavelengths (>740 nm). These features are the consequence of a combination of two processes: the first is a Δ A / A 0 increase for low wavelengths when the transition from GO to rGO occurs (see Fig. 3c ). The second is the well-known wavelength-dependent increase of Δ A / A 0 in water that peaks at 750 nm due to the generation of solvated electrons following multiphoton ionization [33] . The transient absorption spectra, being a combination of these two effects as depicted in Fig. 3c , confirms a GO to rGO transition on the picosecond time scale. 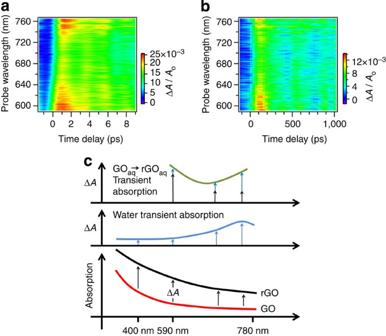Figure 3: Ultrafast spectral changes during reduction. Transient differential absorption spectroscopy of a 2 mg ml−1graphene oxide dispersion in water with a 266 nm pump and white light probe (590–760 nm). Time delays up to (a) 10 ps and (b) 1 ns shown. (c) Sketch of the processes resulting in the transient differential absorption spectra. The contribution of reduction overlaps with the rising transient absorption signal of (W) water with contributions from (rGO) reduced graphene oxide. Figure 3: Ultrafast spectral changes during reduction. Transient differential absorption spectroscopy of a 2 mg ml −1 graphene oxide dispersion in water with a 266 nm pump and white light probe (590–760 nm). Time delays up to ( a ) 10 ps and ( b ) 1 ns shown. ( c ) Sketch of the processes resulting in the transient differential absorption spectra. The contribution of reduction overlaps with the rising transient absorption signal of (W) water with contributions from (rGO) reduced graphene oxide. Full size image Although our results are consistent with the interpretation of solvated electron-mediated reduction, to conclusively rule out the possibility of direct reduction under the described conditions we performed an additional control experiment. A so-called electron scavenger (a species that is well known in the field of radiochemistry) was used to ‘capture’ the solvated electrons thereby removing the source of excess electrons. For this purpose, 0.75% (v/v) acetone was mixed in a 2 mg ml −1 aqueous GO dispersion. Time-resolved differential absorption data ( Fig. 4 ) shows the evolution of the reaction. One can see a significant decrease in the intensity over the whole trace in comparison to a pure GO dispersion. This behaviour demonstrates that solvated electrons, produced in water after ultraviolet excitation, are rapidly quenched in the presence of acetone [37] . As acetone and GO are both present in the solution, a competition takes place for the capture of solvated electrons. The existence of these two reaction pathways diminishes the overall yield of the rGO production ( Fig. 4 ). These results testify that the excess electrons provided by the water ionization are imperative for the ultraviolet photoreduction of GO. 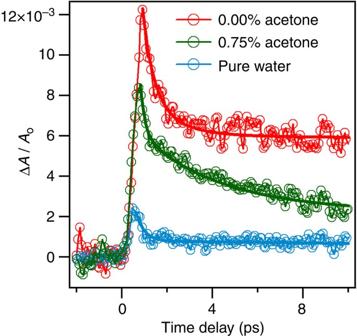Figure 4: Quenching of the reduction by removal of solvated electrons. Transient differential absorption of a 2 mg ml−1graphene oxide (red) without acetone, (green) with 0.75% acetone and (blue) pure water. Figure 4: Quenching of the reduction by removal of solvated electrons. Transient differential absorption of a 2 mg ml −1 graphene oxide (red) without acetone, (green) with 0.75% acetone and (blue) pure water. Full size image To accurately interpret and understand the presented results, it is important to explore the possible reaction pathways leading to the reduction of GO. Because the reaction under consideration is initiated by an intense laser source, one needs to rule out the possibility of a thermally activated process. To estimate the temperature rise of the GO flakes caused by the ultraviolet laser exposure, we consider the illumination volume as a cylinder of radius R and length L , where R is the laser focal radius and L is the cuvette path length. The temperature increase Δ T per laser shot can be conservatively estimated by dividing the energy deposited into the excitation volume by the heat capacity of GO: where p is the fraction of ultraviolet light absorbed by GO, Q is the laser pulse energy and C GO and c GO are the concentration and heat capacity of GO, respectively. The heat capacity is assumed to be similar to that of graphite, and so a value of c GO =2J/gK can be used [38] , [39] . The fraction of absorbed light was found to be p ≈0.43 from the static absorption spectrum, giving a temperature increase of Δ T ≈4.5 K per laser shot. Additionally, possible heat transfer to the bath was not accounted for, and this would serve to decrease the GO temperature. As the sample is continuously refreshed through flow, accumulative heating is excluded. Such a temperature is far below previously reported thermal treatments leading to any observable reduction [18] . A second possible pathway is the direct photoreduction of GO; if occurring such a process would consist of the photoionization of the GO, as ultraviolet light (4.6 eV) is far from any resonant excitation of C–O or C=O bond but near the work function [40] (4.9 eV). However, photoionization would lead to the creation of an electron-hole pair and consequently further oxidize the sample, not reduce it. Based on these arguments, it is unlikely that thermal or direct processes contribute significantly to the reduction. Instead, our results support a final pathway: solvated electron-induced reduction. Such a phenomenon will only happen in a solvent that is able to produce and sustain solvated electrons. Although previous ultrafast optical studies [41] , [42] , [43] , [44] have focused on studying the dynamics of graphene, GO and rGO under various conditions (showing the evolution of valence band electrons after their excitation), it is very important for the reader to notice that what we showed here is the dynamics of a non-reversible chemical reaction (GO→rGO) which is a fundamentally different and so far unobserved process. This work demonstrates that the photoinduced transformation of GO to rGO is an indirect process. The ultrafast nature of this mechanism was revealed by transient absorption spectroscopy with a wide range of wavelengths. It was found that GO is transformed into rGO after the capture of solvated electrons produced by ultraviolet photoionization of the solvent. This sequence of events testifies to the non-thermal nature of the reduction in that it is the chemical potential of the solvated electrons that drives the reduction and not simple heating effects on barrier crossing. A mixture of GO, water and acetone was used to create a competing electron-capture reaction pathway between GO and acetone, hence demonstrating the crucial aspect of the solvent and the indispensable role of the solvated electrons. Our study calls for new investigations of the reduction dynamics of GO in the solid state. Production of aqueous GO dispersions GO flakes were prepared by the Staudenmaier method [12] and characterized by ultraviolet—visible spectroscopy, Raman spectroscopy and XPS. Aqueous dispersions were prepared by mixing GO in ultrapure demineralized, deionized water (18.2 MΩ cm) and sonicating overnight in a sonicator bath (Bandelin Sonorex RK 510, 400 W). Very high loading of GO was required in order to achieve a sufficiently high optical density to give a measurable signal. This high loading (~10 g ml −1 ) led to precipitation of non-exfoliated GO flakes in the prepared dispersion, therefore the supernatant was separated using centrifugation (10 min at 3,000 r.p.m. in a Hermle Z 206 A). The final concentration (~2 mg ml −1 ) of the supernatant was measured by drying a small volume and weighing the resulting GO flakes. Characterization Optical pump–probe experiments were performed in transmission mode with a 1 kHz regenerative femtosecond laser system that provided 50 fs pulses at 800 nm. The 400 nm probe and the 266 nm pump were produced from the harmonics of the fundamental beam using BBO (beta barium borate) nonlinear crystals. The final pulse durations of the pump and probe were about 70 and 90 fs, respectively. The pump and probe were focused on the sample at incident angles of 31° (pump) and 50° (probe) with respect to the surface normal of the sample cell with spot diameters of 220 μm (pump) and 80 μm (probe). The transmission through the sample was detected using a photodiode and a lock-in amplifier after modulating the pump with a 500 Hz optical chopper. The transient absorption spectroscopy measurement used the same geometry except a fibre-coupled Avantes spectrometer was used to measure the transmission and the white light probe was produced by focusing the fundamental into a 2-mm piece of sapphire. The pump power was 800 μW at 500 Hz (1.6 μJ per pulse). The sample was flowed through a ultraviolet fused-silica optical cell with a 1-mm pathlength. The flow rate was on the order of 3 ml min −1 . The static ultraviolet–visible spectra were measured using a Shimadzu UV-2600 spectrophotometer. X-ray photoelectron spectroscopy measurements were performed under ultrahigh vacuum conditions with a base pressure of 5 × 10 −10 mbar in a SPECS GmbH instrument equipped with a monochromatic Mg Kα source (hν=1253.6 eV) and a Phoibos-100 hemispherical analyser. Minute quantity of the GO or RGO suspension were drop casted onto a doped silicon substrate and left to dry in air before transfer to ultrahigh vacuum. Binding energies were corrected using the C–C* at 284.75 eV as reference. Raman spectra were recorded with a Micro-Raman system RM 1000 RENISHAW using a laser excitation line at 532 nm (Nd–YAG) in the range of 1,000–2,000 cm −1 . A power of 1 mW was used with 1 μm focusing spot in order to avoid photodecomposition of the samples. The preparation of the sample was done as for XPS but on a glass substrate. How to cite this article: Gengler, R. Y. N. et al . Revealing the ultrafast process behind the photoreduction of graphene oxide. Nat. Commun. 4:2560 doi: 10.1038/ncomms3560 (2013).